Enrichment of CD56dimKIR+CD57+ highly cytotoxic NK cells in tumour-infiltrated lymph nodes of melanoma patients An important checkpoint in the progression of melanoma is the metastasis to lymph nodes. Here, to investigate the role of lymph node NK cells in disease progression, we analyze frequency, phenotype and functions of NK cells from tumour-infiltrated (TILN) and tumour-free ipsilateral lymph nodes (TFLN) of the same patients. We show an expansion of CD56 dim CD57 dim CD69+CCR7+KIR+ NK cells in TILN. TILN NK cells display robust cytotoxic activity against autologous melanoma cells. In the blood of metastatic melanoma patients, the frequency of NK cells expressing the receptors for CXCL8 receptor is increased compared with healthy subjects, and blood NK cells also express the receptors for CCL2 and IL-6. These factors are produced in high amount in TILN and in vitro switch the phenotype of blood NK cells from healthy donors to the phenotype associated with TILN. Our data suggest that the microenvironment of TILN generates and/or recruits a particularly effective NK cell subset. T-cell-mediated immune responses to melanoma antigens have been documented extensively [1] , [2] . NK cells contribute to anti-tumour immunity, which is traditionally analysed using human peripheral blood NK cells [3] . In contrast, the role of NK cells in the progression of melanoma to lymph node metastasis has not been investigated. We, therefore, set out to analyse and compare NK cell phenotype and responses in tumour-infiltrated lymph nodes (TILN), ipsilateral tumour-free lymph nodes (TFLN) and peripheral blood lymphocytes (PBL) in a cohort of stage III–IV melanoma patients. The NK cells in healthy lymph nodes are predominantly CD56 bright (ref. 1 ). The comparative analysis of the lymphocyte subsets from lymph nodes and autologous peripheral blood reveals a perturbation of NK cell subpopulation frequencies in the TILN where the CD56 dim CD3− NK cells prevail. The phenotype of the NK cells present in the TILN resemble a recently described mature and highly cytotoxic NK subset [4] , [5] . The TILN-associated NK subset is functionally active and mediates a robust anti-melanoma cytotoxicity. Moreover, CXCL8, CCL2 and IL-6 dominate the lymph node–tumour environment and patient’s peripheral blood NK cells indeed express higher amount of CXCR2 and CCR2. Our study reveals an unexpected crosstalk between the tumour niche environment and NK cells and identify a selective anti-melanoma response mediated by CD56 dim CD57+CD69+CCR7+KIR+ NK subset. Frequency and phenotype of NK cells in melanoma patients We found roughly twofold more NK cells within TILN (1.3±0.9% of the total lymphocyte population, n =31) versus TFLN (0.7±0.3%, n =12, P =0.02). We analysed NK cell subsets in blood and lymph nodes by flow cytometry, using the gating strategy depicted in Supplementary Fig. 1 . NK cells can be broadly divided in CD56 dim cytotoxic cells, which represent the majority of NK cells in the blood, and in CD56 bright cytokine producers, which are the most frequent NK cells in lymph nodes [1] . Interestingly, we found that pattern of distribution of these two subsets was significantly perturbed in the blood as well as in the infiltrated lymph nodes of melanoma patients ( Fig. 1a,b ). The mean frequency of NK cells in patients’ peripheral blood (P-PBL) was 5.4±2.0% ( n =10) with a prevalence of the CD56 dim subset (56.5%±17.5) over the CD56 bright subset (43.5±17.5%) ( Fig. 1b ); the latter ratio was significantly different from the one that we and others have found in healthy individuals’ PBL [6] ( Fig. 1b ; H-PBL, CD56 dim =87.8±6.3%; CD56 bright =12.2±6.3%, n =3, P <0.001). As for the lymph nodes, the pattern was now reversed ( Fig. 1b ); the CD56 dim subset prevails in the TILN of all the patients tested (CD56 dim =55.5±21.5%, n =31, CD56 bright =44.5±21.5%, P <0.05) whereas the CD56 bright subset prevailed in TFLN (CD56 dim =31.7±10.8%, n =31, CD56 bright =68.3±10.8%, n =12, P <0.001) just as they do in the lymph nodes of healthy individuals. Thus, NK cell subsets were abnormally distributed in melanoma patients, with the potentially cytotoxic CD56 dim NK cells being underrepresented in patients PBL and overrepresented in TILN. The activation marker CD69 in TILN NK cells was even higher than in peripheral NK cells from both patients and healthy donors ( Fig. 1c , P ≤0.005). 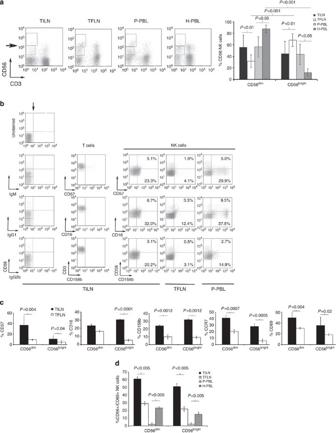Figure 1: Frequency and phenotype of human NK cells in melanoma patients. (a) Representative example (left) for cytofluorimetric analysis of CD56+CD3− NK cell subsets distribution from TILN, TFLN and PBL (P-PBL) in a metastastic melanoma patient in comparison with healthy donor PBL (H-PBL), in the same experimental conditions. Two regions were selected to represent, respectively, CD56brightand CD56dimpopulations. Bar graphs (right) report mean±s.d. of the frequency of CD56dimand CD56brightNK subsets within TILN (black column,n=31) and TFLN (white column,n=12) gated on lymphocytes of all metastatic melanoma patients tested. In parallel, light grey columns show the frequency of CD56dimand CD56brightNK subsets within peripheral blood lymphocytes of patients (P-PBL,n=10) and dark grey columns that of healthy controls (H-PBL,n=3). Statistical analysis is indicated (ANOVA). (b) Expression of CD57, CD16 and CD158b on CD56dimand CD56brightNK cell subsets from TILN, TFLN and P-PBL. Dot plots from one representative patient are presented. The quadrant marker has been set according to the isotype controls; to corroborate the validity of the markers, T cells were used as internal negative control in vertical and the bright/dim boundary in horizontal. The identical quadrant marker has been applied on all the plots. (c) Expression of CD57, CD16, CD158b, CCR7, CD69 on CD56dimand CD56brightNK cell subsets. Bar graphs report mean±s.d. of the percentage of positive cells for each indicated marker in gated NK cells from TILN and TFLN of metastatic melanoma patients (n=12). Statistical analysis is indicated (ANOVA). (d) CD69+ CD56+CD3− NK cell subsets frequencies from TILN (n=31), TFLN (n=12), P-PBL (n=10) and H-PBL (n=3). Values shown are the mean±s.d. of percentages of double positive cells indicated. In all experiments, shownPvalue is calculated by analysis of variance (ANOVA) followed bypost hocBonferroni test. Figure 1: Frequency and phenotype of human NK cells in melanoma patients. ( a ) Representative example (left) for cytofluorimetric analysis of CD56+CD3− NK cell subsets distribution from TILN, TFLN and PBL (P-PBL) in a metastastic melanoma patient in comparison with healthy donor PBL (H-PBL), in the same experimental conditions. Two regions were selected to represent, respectively, CD56 bright and CD56 dim populations. Bar graphs (right) report mean±s.d. of the frequency of CD56 dim and CD56 bright NK subsets within TILN (black column, n =31) and TFLN (white column, n =12) gated on lymphocytes of all metastatic melanoma patients tested. In parallel, light grey columns show the frequency of CD56 dim and CD56 bright NK subsets within peripheral blood lymphocytes of patients (P-PBL, n =10) and dark grey columns that of healthy controls (H-PBL, n =3). Statistical analysis is indicated (ANOVA). ( b ) Expression of CD57, CD16 and CD158b on CD56 dim and CD56 bright NK cell subsets from TILN, TFLN and P-PBL. Dot plots from one representative patient are presented. The quadrant marker has been set according to the isotype controls; to corroborate the validity of the markers, T cells were used as internal negative control in vertical and the bright/dim boundary in horizontal. The identical quadrant marker has been applied on all the plots. ( c ) Expression of CD57, CD16, CD158b, CCR7, CD69 on CD56 dim and CD56 bright NK cell subsets. Bar graphs report mean±s.d. of the percentage of positive cells for each indicated marker in gated NK cells from TILN and TFLN of metastatic melanoma patients ( n =12). Statistical analysis is indicated (ANOVA). ( d ) CD69+ CD56+CD3− NK cell subsets frequencies from TILN ( n =31), TFLN ( n =12), P-PBL ( n =10) and H-PBL ( n =3). Values shown are the mean±s.d. of percentages of double positive cells indicated. In all experiments, shown P value is calculated by analysis of variance (ANOVA) followed by post hoc Bonferroni test. Full size image Maturation and activation markers were measured by multiparametric flow cytometric analysis in TILN, TFLN and PBL. Both CD56 dim and CD56 bright NK cell subsets within TILN showed higher expression of CD57, CD69 and CCR7, whereas CD16 expression was significantly augmented in TILN only in the CD56 bright subset ( Fig. 1d ). The CD57 marker has been recently associated with a late, possibly final stage of NK cell maturation [5] . CD57+ NK cells were 3.4-fold more abundant in TILN (48±17.6%, n =31) than in TFLN (14±4.2%, n =12) ( P =0.002). It should be noted that the intensity of CD57 staining of NK cells in TILN was weaker compared with the CD57+ subpopulation in the blood ( Fig. 1a ). Inhibitory killer-cell immunoglobulin-like receptors (KIRs) control several functions of mature NK cells [7] , [8] . In spite of the marked variability in KIR expression by TILN and TFLN NK cell subsets, the expression of the two inhibitory KIRs stained by the CD158b-specific mAb KIR2DL2 and KIRDL3 was higher on TILN NK cells than on TFLN NK cells ( n =3, P =0.002) ( Fig. 1d ). In line with these data, the intensity of the staining of TILN NK cells by mAbs that recognize KIR3DL2, KIR2DL1/S1, KIR2DL2/L3/S2, KIR2DL1/S1 and CD94 was higher than that of TFLN NK cells in three representative patients (AMM16, 17 and 18, Supplementary Fig. 2a ); the difference was statistically significant ( P ≤0.005, for KIR2D, KIR2DS, KIR3DL and KIR2DL1/S1; P ≤0.05 for CD94) ( Supplementary Fig. 2a,b ). There was also a trend towards a higher expression of activating receptors NKG2D, DNAM-1 and Natural Cytotoxicity Receptors (NCR, also known as NKP30, NKP44 and NKP46) on TILN NK cells in seven metastatic melanoma patients (AMM5, 6, 11, 12, 13, 15 and 16). We have previously reported that NCRs and DNAM-1 are key receptors for NK cell recognition of melanoma cells and, in particular, of melanoma cell lines derived from lymph node metastases; the latter are more susceptible to NK cell recognition because they express higher levels of ligands for NCRs [9] . Together, these results argue in favour of the possibility that TILN is the site where NK cells preferentially enrich and express receptors (KIR, NCR) and markers of maturation (CD57, CD56 dim ) and activation (CD69) suggestive of a more differentiated effector cell phenotype. Moreover, these CD56 dim NK cells expressed the lymph node homing chemokine receptor CCR7 ( Fig. 1d ), suggesting that NK cells actively migrate into the TILN from non-lymphoid tissues and from the circulation. The pattern that we observed can be because of migration of already fully mature CD57+ NK cells to the TILN, or to maturation in situ of immature NK cells migrated from the periphery to TILN. The reduced proportion of CD56 dim cells in the PBL of melanoma patients argues in favour of the former possibility. On the other hand, the low CD57 staining on NK cells in TILN suggests that this subpopulation does not correspond exactly to the CD57 bright NK cells in the blood. In either scenario, our data suggest that TILN might be an important site for NK cell-mediated immunosurveillance against melanoma metastases. Analysis of cytokine milieu in TILN and TFLN To test whether the phenotypical differences between the NK cells resident in TILN and those resident in TFLN were because of different cytokine milieus, we performed transwell co-culture experiments. We observed a strong increment in the percentage of both CD69 and CCR7 expressing cells from TFLN treated with TILN supernatants, reaching very similar levels to TILN NK cells ( Fig. 2a ); this suggests that TILN supernatants contain soluble factors able to convert the phenotype of TFLN NK cells into a phenotype similar to that of TILN NK cells. Thus, we quantified selected cytokines and growth factors in culture supernatants of lymph node-derived cell suspensions from 0 to 96 h. TILN produced more CXCL8 ( Fig. 2b ; P <0.005, n =3), IL-6 and CCL2 than TFLN ( Fig. 2c ) ( P <0.05, n =3). Taken together, these results show that TILN have a different cytokine milieu, which may account for the peculiar NK cell phenotype observed. The expression of CXCL8 and CCL2 chemokines in TILN suspensions might be an early consequence of target cell recognition by NK cells, which has a low threshold for activation [10] . The production of inflammatory cytokines TNFα (tumour necrosis factor alpha) and IFN-γ (interferon gamma) by NK cells, instead, requires stronger activation, which may not be attained in the TILN microenvironment, where tumour and NK cells are exposed to other cytokines and tumour growth factors that may be suppressive. Notably, the autologous melanoma metastasis itself produced detectable amounts of CXCL8, IL-6 and CCL2. To assess the impact of these soluble factors on NK cell phenotype, we treated healthy donors PBL cells with single cytokines or a combination of them ( Supplementary Fig. 3 ). CD56 bright was the only cell subset responsive to the combination of all the three cytokines as it showed an upregulated expression of CD69, CD57, CD16, CD158 and CCR7 ( Fig. 2d ). Similar data were obtained using purified NK cells. 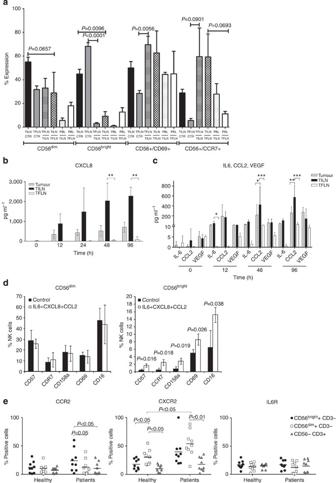Figure 2: Analysis of cytokine milieau in melanoma-infiltrated and tumour-free lymph nodes. (a) Transmissible factors’ influence on CD56 cell subset frequency and CD69 and CCR7 cell surface expression was evaluated in transwell co-cultures. TILN and TFLN samples (n=3) were analysed for CD69 and CCR7 expression within CD56dimand CD56brightNK cell subsets. Each specific bar pattern represents the transwell condition with TFLN, TILN or PBL in the upper chamber of the transwell and TFLN or TILN in the lower one. The bar diagram shows the mean of values±s.d. (analysis of variance (ANOVA),n=3). (b,c) Cytokine production in supernatant of TILN, TFLN and melanoma tumour samples. (b) The histogram reports CXCL8 production by tumour cells (grey column), TILN lymphocytes (black column) and TFLN lymphocytes (white column) as mean±s.d. of three independent experiments. (c) IL-6, CCL2, VEGF release by tumour cells, TILN and TFLN lymphocytes (the results represent mean±s.d. of three separate experiments, ANOVA). Selected statistical analyses are indicated. (ANOVA, *P<0.05, **P<0.01 and ***P<0.001). (d) The combination of IL-6, CXCL8 and CCL2 can influence CD56brightphenotype on CD56+CD3− NK cells derived from peripheral blood of healthy donors. Bars shows the percentage±s.d. of CD56dim(left panel) and CD56bright(right panel) expressing each indicated marker. Results shown are representative of three independent experiments. Statistical analysis is indicated (ANOVA). (e) Frequency of NK and T cell subsets (CD56bright+CD3−; CD56dim+CD3−; CD56−CD3+) expressing the CXCL8 receptor (CXCR2), CCL2 receptor (CCR2) and IL-6 receptors in healthy donors (n=8) and melanoma patients peripheral blood (n=9). Each dot represents a different patient or healthy donor. Bars represent mean values. Statistical analysis is indicated (ANOVA). VEGF, vascular endothelial growth factor. Figure 2: Analysis of cytokine milieau in melanoma-infiltrated and tumour-free lymph nodes. ( a ) Transmissible factors’ influence on CD56 cell subset frequency and CD69 and CCR7 cell surface expression was evaluated in transwell co-cultures. TILN and TFLN samples ( n =3) were analysed for CD69 and CCR7 expression within CD56 dim and CD56 bright NK cell subsets. Each specific bar pattern represents the transwell condition with TFLN, TILN or PBL in the upper chamber of the transwell and TFLN or TILN in the lower one. The bar diagram shows the mean of values±s.d. (analysis of variance (ANOVA), n =3). ( b , c ) Cytokine production in supernatant of TILN, TFLN and melanoma tumour samples. ( b ) The histogram reports CXCL8 production by tumour cells (grey column), TILN lymphocytes (black column) and TFLN lymphocytes (white column) as mean±s.d. of three independent experiments. ( c ) IL-6, CCL2, VEGF release by tumour cells, TILN and TFLN lymphocytes (the results represent mean±s.d. of three separate experiments, ANOVA). Selected statistical analyses are indicated. (ANOVA, * P <0.05, ** P <0.01 and *** P <0.001). ( d ) The combination of IL-6, CXCL8 and CCL2 can influence CD56 bright phenotype on CD56+CD3− NK cells derived from peripheral blood of healthy donors. Bars shows the percentage±s.d. of CD56 dim (left panel) and CD56 bright (right panel) expressing each indicated marker. Results shown are representative of three independent experiments. Statistical analysis is indicated (ANOVA). ( e ) Frequency of NK and T cell subsets (CD56 bright +CD3−; CD56 dim +CD3−; CD56−CD3+) expressing the CXCL8 receptor (CXCR2), CCL2 receptor (CCR2) and IL-6 receptors in healthy donors ( n =8) and melanoma patients peripheral blood ( n =9). Each dot represents a different patient or healthy donor. Bars represent mean values. Statistical analysis is indicated (ANOVA). VEGF, vascular endothelial growth factor. Full size image The expression of the receptors for CXCL8, CCL2 and IL-6 was compared in healthy donors and melanoma patient’s peripheral blood NK cells. The frequency of CXCR2 was significantly higher in the CD56 dim compartment in patients’ peripheral blood with respect to healthy donors. There was a trend towards higher expression of both CXCR2 and CCR2 in the CD56 bright subset in patients’ PBL. Noteworthy, no differences were found in T cells compartment between healthy donors and patients. The frequencies of CXCR2 and CCR2 expressing NK cells were higher than T cells with these receptors in patients' peripheral blood. However, only the CD56 dim CXCR2 expressing subset and CD56 bright CCR2 reached the statistical significance ( Fig. 2e ). Therefore, it is conceivable to propose that the presence of metastatic cells lead to a cytokine environment in the patients’ lymph node that is dominated by CXCL8, CCL2 and IL-6 ( Fig. 2b ). These soluble factors may induce in situ maturation of CD56 bright CD3− NK cells to become more mature and cytotoxic CD57+KIR+CD69+CCR7+ NK cells ( Fig. 2d ). Moreover, CXCL8 and CCL2 produced by metastatic lymph nodes may recruit CXCR2+/CCR2+ cells among both subsets of circulating CD56 bright and CD56 dim NK cells ( Fig. 2e ). NK cells cytotoxicity from tumour-infiltrated lymph nodes To directly quantify the anti-tumour activity of patients’ NK cell subsets, we measured NK cell cytotoxicity against patients’ autologous melanoma cells after short-term cultures. We included NK cells isolated from patients’ TILN, TFLN and PBL, as well as NK cells isolated from healthy donors' PBL. TILN NK cells showed the highest and TFLN NK cells the lowest cytotoxic activity ( Fig. 3a,b ). Altogether, these data demonstrate that autologous TILN-derived NK cells kill lymph node metastatic melanoma cells more efficiently than autologous TFLN- and PBL-derived NK cells ( P ≤0.005, n =6), or allogeneic PBL-derived NK cells from healthy donors ( P ≤0.005, n =4). To confirm the cytotoxic potential of NK cells in vitro , we used a degranulation assay based on the expression of CD107a. We measured basal CD107a surface expression directly after explanting TILN and TFLN of five melanoma patients (AMM17, 18, 19, 20, 21). In all the patients tested, the expression of CD107a was higher on NK cells from TILN, particularly within the CD56 dim cells ( P =0.012) and the CD57+ NK cells ( P =0.005; Fig. 3c ). We also measured degranulation in response to K562 erythroleukemia cells, the gold standard target for NK cells. Interestingly, only TILN NK cells were clearly activated to degranulate by K562 pulsing, while the TFLN NK cells were unresponsive ( Fig. 3d ). To assess whether these highly cytotoxic TILN CD57+CD56+ NK cells maintain proliferative potential, we measured the expression of Ki67, a marker of cycling cells. CD57+CD56+ NK cells contained sixfold more Ki67+ cycling cells (60.1%±13.4) than CD57-CD56+ NK cells (10.4% ±10.2), thus they can proliferate ( Fig. 3e ). 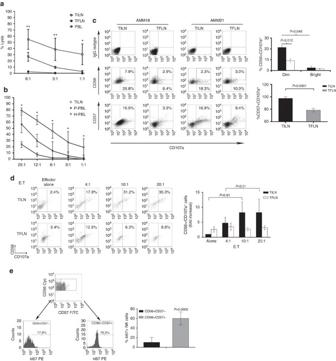Figure 3: NK cells from tumour-infiltrated lymph nodes have strong cytotoxic potential. (a,b) Cytotoxicity of NK cells against autologous melanoma cell lines. The graph reports the mean percentage specific lysis ±s.d. of at least three individual representative experiments performed at the indicated Effector:Target (E:T) ratios. (a) The figure compares killing by autologous NK cells isolated from patients’ TILN (circle symbol) and TFLN (black square) or allogenic NK cells isolated from healthy donors’ PBL (H-PBL, black triangle). (b) Comparison between cytotoxicity of autologous NK cells isolated from TILN (circle symbol,n=6), patients’ PBL (P-PBL, black triangle,n=4) and allogenic NK cells isolated from healthy donors’ PBL (H-PBL, white triangle,n=4). Selected statistical analyses are indicated. (ANOVA, *P<0.05 and **P<0.01). (c) Basal CD107a surface expression on TILN- and TFLN-NK cells from two representative (AMM18 and AMM21) patients, as assessed by FACS analysis. Numbers in dot plots indicate the percentage of CD107a positive cells within CD56dimand CD56brightNK subsets (upper panels) or alternatively within CD57+CD56+ NK cells (lower panels). The dot plot quadrants are set according to the isotype IgG control for TILN and TFLN as shown in the figure. In the CD56 dot plots, two additional regions identify bright and dim NK cell subsets. The bar diagrams (right) refer to the mean of values±s.d. of experiments performed in five metastatic melanoma patients (ANOVA). (d) Two representative metastatic melanoma patients (AMM17 on the left and AMM20 on the right) FACS analysis of the CD107a mobilization assay gating on CD56+CD3− TILN and TFLN NK cells after K562 pulsing at different E:T ratios. Quadrants are drawn according to the IgG isotype control for TILN and TFLN, as shown. The bar diagram (right) shows the mean of values±s.d. (n=4) expressed as fold increase of CD107a expression in target pulsed NK cells over NK cells alone. (e) Ki67 intracellular staining of TILN CD57+CD56+ NK cells. The bar diagram (right) shows the mean of values±s.d. (n=5). Figure 3: NK cells from tumour-infiltrated lymph nodes have strong cytotoxic potential. ( a , b ) Cytotoxicity of NK cells against autologous melanoma cell lines. The graph reports the mean percentage specific lysis ±s.d. of at least three individual representative experiments performed at the indicated Effector:Target (E:T) ratios. ( a ) The figure compares killing by autologous NK cells isolated from patients’ TILN (circle symbol) and TFLN (black square) or allogenic NK cells isolated from healthy donors’ PBL (H-PBL, black triangle). ( b ) Comparison between cytotoxicity of autologous NK cells isolated from TILN (circle symbol, n =6), patients’ PBL (P-PBL, black triangle, n =4) and allogenic NK cells isolated from healthy donors’ PBL (H-PBL, white triangle, n =4). Selected statistical analyses are indicated. (ANOVA, * P <0.05 and ** P <0.01). ( c ) Basal CD107a surface expression on TILN- and TFLN-NK cells from two representative (AMM18 and AMM21) patients, as assessed by FACS analysis. Numbers in dot plots indicate the percentage of CD107a positive cells within CD56 dim and CD56 bright NK subsets (upper panels) or alternatively within CD57+CD56+ NK cells (lower panels). The dot plot quadrants are set according to the isotype IgG control for TILN and TFLN as shown in the figure. In the CD56 dot plots, two additional regions identify bright and dim NK cell subsets. The bar diagrams (right) refer to the mean of values±s.d. of experiments performed in five metastatic melanoma patients (ANOVA). ( d ) Two representative metastatic melanoma patients (AMM17 on the left and AMM20 on the right) FACS analysis of the CD107a mobilization assay gating on CD56+CD3− TILN and TFLN NK cells after K562 pulsing at different E:T ratios. Quadrants are drawn according to the IgG isotype control for TILN and TFLN, as shown. The bar diagram (right) shows the mean of values±s.d. ( n =4) expressed as fold increase of CD107a expression in target pulsed NK cells over NK cells alone. ( e ) Ki67 intracellular staining of TILN CD57+CD56+ NK cells. The bar diagram (right) shows the mean of values±s.d. ( n =5). Full size image Frequency of CD57+CD56 dim NK cells in TILN and prognosis The peculiar phenotype of TILN NK cells and their surprisingly high cytotoxic activity against autologous melanoma cells, prompted us to investigate whether the presence of the CD57+CD56 dim subset in TILN would correlate with clinical outcome. The ratios between CD57+CD56 dim and CD57+CD56 bright cells, normalized on the total NK cells percentage in TILN, showed considerable variability among the 20 melanoma patients’ TILN investigated, distributing over a range between 1.0 and 16.9 ( Fig. 4a and Supplementary Table 2 ). We thus divided the patients into two groups, one with a ≥6 ratio and the other one with a <6 ratio. Since patients with higher ratio mainly belong to stage III, we stratified the patients according to disease stage ( Fig. 4b ), and found a trend towards association between overall survival and NK ratio within stage III patients. 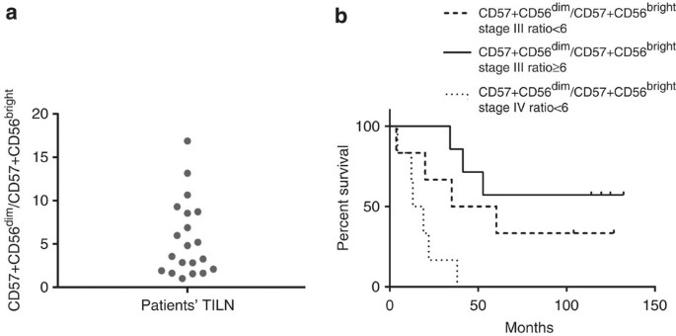Figure 4: Stratifying by stages patients' survival in groups with high or low frequency of CD56dimCD57+ NK cells in tumour-infiltrated lymph nodes. (a) CD57+CD56dim/CD57+CD56brightratio was calculated as a proportion of total NK cell frequency in the melanoma-infiltrated lymph nodes (TILN) of each metastastic melanoma patient. (b) Kaplan–Meier survival curves in seven patients with CD57+CD56dim/CD57+CD56brightratio ≥6 (continuous line), six patients with CD57+CD56dim/CD57+CD56brightratio <6 stage III (dashed line) and with six patients CD57+CD56dim/CD57+CD56brightratio <6 in stage IV (dotted line). The curves were compared with log-rank test (P=0.004) and a test for trend (P=0.00068). Figure 4: Stratifying by stages patients' survival in groups with high or low frequency of CD56 dim CD57+ NK cells in tumour-infiltrated lymph nodes. ( a ) CD57+CD56 dim /CD57+CD56 bright ratio was calculated as a proportion of total NK cell frequency in the melanoma-infiltrated lymph nodes (TILN) of each metastastic melanoma patient. ( b ) Kaplan–Meier survival curves in seven patients with CD57+CD56 dim /CD57+CD56 bright ratio ≥6 (continuous line), six patients with CD57+CD56 dim /CD57+CD56 bright ratio <6 stage III (dashed line) and with six patients CD57+CD56 dim /CD57+CD56 bright ratio <6 in stage IV (dotted line). The curves were compared with log-rank test ( P =0.004) and a test for trend ( P =0.00068). Full size image Although suggestive of a potential role for lymph node NK cells in clinical outcome, this association must be considered as a preliminary observation, to be tested in a much larger cohort to assess whether it is an independent variable. In contrast, there was no such pattern when patients were grouped according to the frequencies of CD57+CD8+CD3+ cytotoxic T cells ( Supplementary Fig. 5 ) or Foxp3+CD25+CD3+ T regulatory cells ( Supplementary Fig. 6 ). The differences in survival cannot be explained by novel therapies for metastatic melanoma such as BRAF inhibitors and anti-CTLA-4 or PD1 monoclonal antibodies, since the patients studied here were diagnosed before the introduction of these treatment protocols. We noted that male patients dominated in the group with <6 ratio (10 males versus two females) but not in the group with >6 ratio (three males versus three females), and males have been reported to have a worse prognosis in metastatic melanoma [11] . We, therefore, cannot exclude gender as a contributing factor in the clinical outcome ( Supplementary Table 1 ). Experimental evidence supports the notion that peripheral blood CD56 bright NK cells give rise to CD56 dim NK cells, which can be further subdivided into subsets on the basis of surface markers and function. CD57 expression is acquired at later stages and marks terminally differentiated cells with high cytolytic activity but very low proliferative potential [5] , [6] , [12] . Under physiological conditions, the NK cell population in lymph nodes is dominated by CD56 bright cells. We found a striking reversed pattern in tumour-infiltrated lymph nodes where most NK cells are CD56 dim CD57+. These cells express activation markers and are highly cytotoxic against autologous melanoma cell lines. In view of these findings, the ratio between the CD57+CD56 dim and the CD57+CD56 bright , normalized on the total NK cell percentage in TILN, could represent a valid index of terminal differentiation toward fully competent and highly cytotoxic NK cells. It is remarkable that despite the presence of T reg cells ( Supplementary Fig. 4 ), these KIR+CD57+ NK cells are activated, as demonstrated by the expression of CD69 and their ability to readily degranulate. The high functional activation status of TILN NK cells can even be further increased by ex vivo exposure to tumour cells such as K562 cells, despite the possible tolerogenic environment. However, it should be noted that the TILN milieu is characterized by considerable IL-6 production ( Fig. 2b ), known to drive CD4 T-cell differentiation away from T reg function even in the presence of TGF-β [13] . Noteworthy, melanoma metastases produce CXCL8 (ref. 14 ) and the senescent melanoma cells secrete IL-6, CCL2 and CXCL8 (ref. 15 ). The serum concentration of CXCL8 increases during melanoma progression [16] . Thus, NK cells may be specifically recruited from the blood to the melanoma-infiltrated lymph nodes using the combination of receptors that facilitate homing (CCR7 and CXCR2) and tumour targeting (CXCR2 and CCR2). The described results suggest that the ratio between CD56 dim CD57+and CD56 bright CD57+ cells in TILN is biologically important and this preliminary observation should be further explored as a prognostic marker in metastatic melanoma. One possible mechanistic/causal scenario that emerges from this observation is that during the progression of malignant melanoma to lymph node metastasis, CD56 dim CD57+ NK cells become enriched in infiltrated lymph nodes, either by selective recruitment or by expansion (or a combination of the two). These NK cells then act to limit further spread. It is, however, also possible that the differential reactivity patterns in the TILN represent consequence rather than cause of differential tumour progression. For example, association with prognosis might be explained by the ability of particularly aggressive tumours to prevent the enrichment of the fully differentiated NK cell subset. These and other aspects of lymph node NK cell reactivity would be interesting to analyze further in a larger cohort of patients. To our knowledge, this is the first report demonstrating that CD56 dim CD57+NK cells can be found in lymph nodes. It will be interesting to investigate how this subpopulation relates to ‘memory’ NK cells that expand after CMV infection in mice and humans [17] , [18] . Besides shedding light on the role of NK cells in tumour protection, our data suggest that TILN NK cells should be considered as interesting candidate for the design of new adoptive immunotherapy protocols. Lymph nodes explanted during common clinical practice may be a good source of proliferating and highly cytotoxic NK cells that can be expanded ex vivo and subsequently administered to patients. Isolation of lymphocytes and melanoma cell cultures Lymphocytes and melanoma cells were isolated from surgically removed tumour-invaded lymph nodes (TILN) and ipsilateral tumour-free lymph nodes (TFLN) of AJCC stage IIIc or IV melanoma patients. Patients were admitted to Fondazione IRCCS Istituto Nazionale dei Tumori, Milan, Italy. Patients had no history of previous chemotherapy or immunotherapy. All the lesions were histologically confirmed to be cutaneous malignant melanomas. Written informed consent was obtained from all patients in accordance with the Declaration of Helsinki to the use of human biological samples for research purposes. Lymphocytes from TILN of 38 patients (named with the acronym AMM and numbered from 1 to 56), TFLN and melanoma cells from TILN, were isolated by mechanical disaggregation of surgical specimens. Briefly, tumour specimens were placed in RPMI 1640 (Lonza Verviers, Belgium) supplemented with antibiotics, such as penicillin and streptomycin (Lonza) and minced into 1–2 mm 3 fragments by surgical scalpels. Further tissue disaggregation was achieved by forcing fragments through a metallic mesh with the aid of a sterile syringe plunger. After centrifugation, the cell suspension was treated with trypsin (Lonza) and DNAase (Sigma) for 2 min at room temperature to remove dead cells. After two washes and centrifugation, different aliquots of the cell suspensions were used for cryopreservation, for deriving tumour cell cultures and for isolation of lymphocytes. Melanoma cell lines were established by culture of cell suspensions in 25 cm 2 tissue flasks in RPMI 1640 supplemented with 2% glutamine (200 mM, Invitrogen), penicillin (100 U ml −1 ) and streptomycin (100 μg ml −1 ) and 10% heat-inactivated fetal calf serum (Biological Industries), at 37 °C in humidified CO 2 atmosphere. Melanoma cell lines were routinely tested for the absence of Mycoplasma contamination by a PCR-based kit (PromoCell). SP11-763.74 (ref. 19 ) and SP11-TP61.5 (ref. 20 ) mAbs that recognize specific melanoma markers were used to validate histologically primary melanoma cell lines derived from individual patients. The human melanoma metastatic cell lines were grown for not more than nine to ten in vitro passages. Lymphocytes from TILN-derived cell suspensions were isolated by Ficoll-Paque (Biopaque) gradient separation. Isolation of NK cells from short-term TILN and TFLN cultures NK cells were purified from TILN and TFLN cell suspensions in selected experiments, using the NK cell Isolation kit negative selection and VarioMACS (Miltenyi Biotec) according to the manufacturer’s instructions for the depletion of non-NK cells. Briefly, after thawing, TILN and TFLN cell suspensions in RPMI 1640 medium were cultured overnight at 37 °C in a 5% CO 2 -humidified atmosphere. After a preliminary passage through a Ficoll column (Biopaque) to remove debris and dead cells, the purity of NK cell preparations, determined by cytofluorimetric analysis, was >95%. Freshly enriched NK cells were suspended in Iscove’s Modified Dulbecco’s culture medium (IMDM, Life Technology) supplemented with penicillin (100 IU ml −1 ) and streptomycin (100 μg ml −1 ), 10% FBS (Invitrogen). PBL were isolated from blood of patients with melanoma or of healthy donors by density gradient centrifugation over Ficoll-Paque (Biopaque). Antibodies Q66 (KIR3DL2)/IgM (at 1:5 dilution), Z27 (KIR3DL1/S1)/IGg1 (at 1:10 dilution), GL183 (KIR2D2/3/S2)/IgG1 (at 1:20 dilution), XA185 (CD94)/IgG1 (at 1:20 dilution), Z 270 (NKG2A) IgG1 (at 1:5 dilution) supernatants produced in our laboratory (A.M.). FITC-anti-CD57/IgM (322306 at a 1:100 dilution), PE-anti-CD57/IgM (322312 at a 1:100 dilution), PerCP/Cy5.5–CD3/IgG1 (344807 at a 1:100 dilution) PE-antiKi67/IgG1 (350503 at a 1:50 dilution), PE/Cy5 anti-human CD56/IgG2a (304608 at a 1:100 dilution), APC-anti-CD3/IgG2a (317317 at a 1:100 dilution), PE-antiFoxp3 /IgG1(320007 at a 1:100 dilution), PE-antiNKp44/IgG1 (325108 at a 1:100 dilution), PE-antiNKp30 IgG1 (325208 at a 1:100 dilution), PE-antiNKp46 IgG1 (331908 at a 1:100 dilution), PE-antiDNAM1/IgG1( 338305 at a 1:100 dilution) and PE-antiNKG2D/IgG1(320806 at a 1:200 dilution), PE-antiCCR7/IgG2a (353204 at a 1:100 dilution), PE-antiCD16/IgG1 (302008 at a 1:300 dilution), FITC-antiCD69/IgG1 (310904 at a 1:100 dilution) were from BioLegend. FITC-anti-CD3/IgG1 (11-0036 at a 1:100 dilution) and APC-anti-CD3/IgG1 (11-0036-42 at a 1:100 dilution) were from eBioscience. PE-Cy7-anti-CD56/IgG1 (560916 at a 1:100 dilution), PE-CD69/IgG1 (341652 1:50 dilution) and FITC-CD158b/IgG2b (559784 at 1:50 dilution) were from BD Pharmingen. For the cytokines receptors staining on patients and healthy donor lymphocytes, the followed antibodies were used: APC-antiCD126 (IL-6R)/IgG1 (cod.562090 at 1:50 dilution), APC-antiCD182 (CXCR2)/IgG1 (cod.551127 at 1:10 dilution), APC-antiCD192 (CCR2)/IgG2b (cod.558406 at 1:10 dilution) from Miltenyi Biotec, and 7AAD Staining Solution for the cell viability from BD Pharmingen. Flow cytometry analysis Briefly, 2 × 10 5 cells from the total LN suspension were stained with the indicated antibodies followed by flow cytometric analysis. In the indirect staining method, the cells were first incubated with an appropriate primary mAb followed by FITC (Sigma) conjugated goat anti-mouse secondary antibody. In all experiments, the isotype-matched controls were used to set up the negative values. Cells were fixed in 1% formaldehyde for data analysis. Sample fluorescence was measured by the fluorescence-activated cell sorter FACSCalibur apparatus (Becton Dickinson) and data were analysed by using the Cell-Quest software (Becton Dickinson). For intracellular staining to investigate the percentage of T reg cell, cell pellets were resuspended in phosphate-buffered saline (PBS) with 2% FBS and stained with fluorochrome-conjugated anti-CD4, then fixed with 3% formaldehyde (Sigma) in PBS, permeabilized with PBS with 2% FBS and 0.5% saponin (Sigma), and stained with PE-antiFoxp3 /IgG1. For Ki67 staining, BD Cytofix/Cytoperm kit was used, according to manufacturer’s instructions. Briefly, cell pellets were resuspended in PBS with 2% FBS and surface stained with fluorochrome-conjugated anti-CD56, anti-CD57 and anti-CD3, then fixed, permeabilized and intracellularly stained with PE-Ki67/IgG1. In the direct staining for the cytokines receptors, cells were first incubated with human serum for 15 min and then acquired by a FACS Canto II apparatus (Becton Dickinson). The data were analysed by Flow-Jo version 7.6.4 software analysis. Microarray cytokine assay For cytokine profile analysis, TILN, TFLN and tumour samples of AMM 8,9,16 metastatic melanoma patients were thawed and cultured with complete RPMI 1640 medium. Then 1,000 μl of culture supernatant were removed at 0, 12, 24, 48, 96 h time points and analysed by biochip array analyser with the RANDOX cytokine and growth factors array (CTK) microarray kit, for the simultaneous quantification of interleukin-2 (IL-2), IL-4, IL-6, CXCL8, IL-10, vascular endothelial growth factor, IFN-γ, TNFα, IL-1α, IL-1β, monocyte chemoattractant protein-1 and epidermal growth factor. This assay was performed following the manufacturer’s recommended procedure. Beads were read on the Bio-Plex suspension array system. Data were analysed using Bio-Plex manager software with 5PL curve fitting. The limit of detection for this assay is ≈10 pg ml −1 (based on detectable signal±2 s.d. above background). TGF-β production was evaluated by a specific ELISA kit following manufacturer’s instructions (R&D Systems and Biosource International). Cytotoxicity assay Purified NK cells from TILN, TFLN and PBL of melanoma patients or healthy donors were cultured for 48 h in the presence of 200 IU of IL-2 (Chiron) than used as effectors against related metastatic melanoma in vitro established tumour cells using the fluorescent carboxy-Fluorescein Diacetate c’FDA NK assay. Briefly, the target cells were labelled with c’FDA (Molecular Probes). Target cells were mixed with effector cells at different E:T ratios for 3 h in 200 μl of RPMI 1640 medium at 37 °C in a humidified 5% CO 2 incubation. The specific lysis of target cells was calculated as follows: % specific lysis=(CT−TE/CT) × 100, (where CT=mean number of fluorescent target cells in control tubes and TE=mean number of fluorescent cells in target+effectors tubes). CD107a mobilization assay after K562 pulsing Freshly enriched lymphocytes from TILN and TFLN cell suspension of metastatic melanoma patients were cultured at 37 °C in 5% CO 2 to different (4:1, 10:1 and 20:1) effector:target ratio with K562 (ATCC) in the presence of PE-conjugated CD107a/IgG1 antibody (BD Pharmingen) in U-bottom 96-well plates. After 1 h, Brefeldin A (5 μg ml −1 , Sigma) was added to cultures for an additional 3 h of incubation. At this time, cells were collected, washed with PBS with 2% fetal bovine serum (FBS) stained with anti-CD56 PE-Cy5 (Beckman-Coulter-Immunotech), anti-CD3 FITC (Beckman-Coulter-Immunotech) or alternatively with anti-CD3 APC (BD Pharmingen) and analysed by flow cytometry. Statistical analysis Data obtained from multiple experiments are calculated as mean±s.d. and analysed for statistical significance using the two-tailed Student’s t -test, for independent groups, or analysis of variance followed by Bonferroni correction for multiple comparisons. P values <0.05 were considered statistically significant. We analysed survival time after surgery in 20 cancer patients. We considered tumour stage (III and IV) and the CD57+CD56 dim /CD57+CD56 bright ratio (ratio <6 and ratio ≥6) as potential predictors. The value 6 of the ratio was chosen because it was the best discriminatory cut-off value for survival. We obtained survival curves with the Kaplan–Meier product-limit estimator. We tested the trend in survival for differences between groups with the log-rank test. Trend in survival across groups of patients was analyzed by testing the coefficient associated with the group entered as a numeric variable in a Cox regression model. We verified proportionality of the hazards with Schoenfeld’s residuals. We tested the association between stage and ratio with the Fisher’s exact test. Statistical computations were done using the graphPad Prism 5.0 software for Windows; the analyses were performed with Stata version 13 (Statacorp, College Station, TX, USA). How to cite this article: Ali, T. H. et al. Enrichment of CD56 dim KIR+CD57+ highly cytotoxic NK cells in tumour-infiltrated lymph nodes of melanoma patients. Nat. Commun. 5:5639 doi: 10.1038/ncomms6639 (2014).